FeOx-supported platinum single-atom and pseudo-single-atom catalysts for chemoselective hydrogenation of functionalized nitroarenes The catalytic hydrogenation of nitroarenes is an environmentally benign technology for the production of anilines, which are key intermediates for manufacturing agrochemicals, pharmaceuticals and dyes. Most of the precious metal catalysts, however, suffer from low chemoselectivity when one or more reducible groups are present in a nitroarene molecule. Herein we report FeO x -supported platinum single-atom and pseudo-single-atom structures as highly active, chemoselective and reusable catalysts for hydrogenation of a variety of substituted nitroarenes. For hydrogenation of 3-nitrostyrene, the catalyst yields a TOF of ~1,500 h −1 , 20-fold higher than the best result reported in literature, and a selectivity to 3-aminostyrene close to 99%, the best ever achieved over platinum group metals. The superior performance can be attributed to the presence of positively charged platinum centres and the absence of Pt–Pt metallic bonding, both of which favour the preferential adsorption of nitro groups. Functionalized anilines are industrially important and valuable intermediates for a variety of agrochemicals, pharmaceuticals, dyes and pigments [1] . Currently, the commercial production of functionalized anilines mainly uses non-catalytic reduction of the corresponding nitroarenes using stoichiometric reducing agents such as sodium hydrosulfite, iron, tin or zinc in ammonium hydroxide [2] . Such processes, however, have serious environmental issues. In this context, there is a great need to search for an environmentally benign and highly efficient method to produce functionalized anilines. Catalytic hydrogenation with supported metal catalysts is the preferred choice [3] . Nevertheless, when one or more reducible groups (for example, C=C, C≡C, C=O, C≡N and so on) are present in a nitroarene molecule, the chemoselective hydrogenation of the nitro group has been a grand challenge. In some cases, through modification of transition metal with well-chosen additives, for example, Pt/C-H 3 PO 2 -VO(acac) 2 and Pt-Pb/CaCO 3 -FeCl 2 - n Bu 4 NCl, chemoselective reduction of nitroarenes was obtained at the expense of activity [4] . Moreover, the addition of soluble metal salts still causes environmental problems. Therefore, the development of true heterogeneous catalysts without the use of any organic/inorganic additives is highly desirable. IB-group metal catalysts, especially supported Au and Ag nanoparticle catalysts, have been reported to show excellent chemoselectivity for the hydrogenation of a variety of substituted nitroarenes [5] , [6] , [7] , [8] , [9] . However, the intrinsically poor capability of IB-group metals for H 2 activation renders them at least one order of magnitude less active than the Pt-group metals. To enhance the activity of IB-group metals, delicate control of metal-support interactions [10] , [11] , [12] , [13] , [14] or alloying with a small amount of Pt-group metals [15] , [16] was tested. However, the achieved chemoselectivity of these catalysts was not satisfactory. Very recently, noble metal-free catalysts based on cobalt– or iron–phenanthroline complexes have been developed for the chemoselective hydrogenation of nitroarens, with excellent chemoselectivities for numerous structurally diverse substrates [17] , [18] , but similar to the IB-group metals they require relatively demanding reaction conditions, for example, long reaction time (more than 12 h), high temperature (120 °C) and high H 2 pressure (50 bar). The chemoselectivity to the hydrogenation of nitro groups arises from the preferential adsorption of nitro groups on the specific sites of metal nanoparticles or the support [13] , [14] . Although the hydrogenation of nitro groups over metal nanoparticles appears to be size insensitive, the hydrogenation of C=C and C≡C groups is indeed highly sensitive to the particle size, with the reaction rate usually increasing with increasing metal particle size [19] . Accordingly, by reducing the particle size of Pt-group metals and by tuning the metal–support interactions, Corma et al. [20] achieved high chemoselectivity (90%–95%) over Pt/TiO 2 , Pt/C, Ru/TiO 2 and even Ni/TiO 2 catalysts while maintaining a high activity. The lowest limit of downsizing metal particles is to disperse the metal as exclusively isolated single atoms, which we previously denoted as ‘single-atom catalyst (SAC)’ [21] . The SAC has exhibited superior activity in CO oxidation [22] , [23] , water–gas shift reaction [24] , [25] , [26] , methane conversion [27] and other important reactions [28] , [29] , [30] . On account of the uniform geometry of single atoms and their good capability for H 2 dissociation [31] , it is expected that the SAC may have superior performance in selective hydrogenation reactions. In this study we report that FeO x -supported Pt single-atom and pseudo-single-atom structures are extremely active, chemoselective and recyclable for the hydrogenation of a variety of functionalized nitroarenes. More importantly, characterizations by aberration-corrected high-angle annular dark-field scanning transmission electron microscopy (HAADF-STEM) and X-ray absorption fine structure spectroscopy (XAFS) reveal that the pseudo-single-atom structure is composed of a few to tens of atoms, which are loosely and randomly associated with each other but do not form strong Pt–Pt metallic bonding, resembling the structure and function of isolated single atoms. For the chemoselective hydrogenation of 3-nitrostyrene, the turnover frequency (TOF) of the SAC and pseudo-SACs reaches as high as ~1,500 h −1 , 20-fold higher than that of the best catalyst reported in literature (Pt/TiO 2 ) [15] . Furthermore, the selectivity toward 3-aminostyrene is close to 99%, again the best result ever achieved over Pt-group metals. HAADF-STEM characterization The series of Pt/FeO x catalysts were prepared by co-precipitation at 50 °C with H 2 PtCl 6 and Fe(NO 3 ) 3 as the metal precursors and Na 2 CO 3 as the precipitation agent [22] . The resultant precipitate was filtered, washed thoroughly with deionized water, dried at 60 °C overnight, calcined in air at 400 °C and reduced with 10% H 2 /He at 200 °C or 250 °C for 30 min. By varying the amount of Pt loading and changing the reduction temperature, the dispersion of Pt metal was finely tuned with their morphologies varying from isolated single atoms, loosely associated ensembles, subnanometre clusters to three-dimensional (3D) nanoparticles. 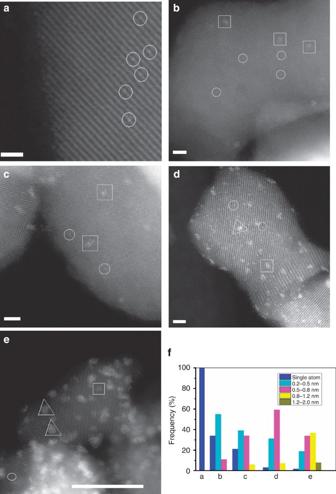Figure 1: HAADF-STEM images and histogram of size distributions. (a) 0.08%Pt/FeOx-R200. Scale bar, 1 nm. (b) 0.08%Pt/FeOx-R250. Scale bar, 2 nm. (c) 0.31%Pt/FeOx-R250. Scale bar, 2 nm. (d) 0.75%Pt/FeOx-R250. Scale bar, 2 nm. (e) 4.30%Pt/FeOx-R250. Scale bar, 10 nm. (f) Histogram of size distributions. The circles, squares and triangles in the figures represent the single atoms, 2D rafts and 3D clusters/particles, respectively. Figure 1 presents the representative HAADF-STEM images of the freshly reduced catalysts. When the Pt loading was 0.08 wt% with a reduction temperature of 200 °C (0.08%Pt/FeO x -R200), all the Pt species existed exclusively as isolated single atoms; neither subnanometre clusters nor nanoparticles were detected ( Fig. 1a ; for more images, see Supplementary Fig. 1 ), which is in accordance with our previous observations [22] . On the other hand, when the 0.08 wt% Pt/FeO x catalyst was reduced at a slightly higher temperature, for example, 250 °C or above, clustering of single atoms occurred and very small clusters composed of loose and random ensembles of several to tens of atoms, with dimensions <0.8 nm, were formed ( Fig. 1b and Supplementary Fig. 2 ). Based on the brightness variations of these clusters in HAADF images and by comparing their intensities with those of the single atoms, we concluded that most of these subnanometre clusters possessed a two-dimensional (2D) raft-like morphology, suggesting the occurrence of strong metal–support interactions [32] . However, with a higher Pt loading (0.31–4.30 wt%) and a reduction temperature at 250 °C, 3D nanoparticles with sizes of 1–2 nm were found to co-exist with the 2D rafts and single atoms ( Fig. 1c–f and Supplementary Figs 3–5 ). Figure 1: HAADF-STEM images and histogram of size distributions. ( a ) 0.08%Pt/FeO x -R200. Scale bar, 1 nm. ( b ) 0.08%Pt/FeO x -R250. Scale bar, 2 nm. ( c ) 0.31%Pt/FeO x -R250. Scale bar, 2 nm. ( d ) 0.75%Pt/FeO x -R250. Scale bar, 2 nm. ( e ) 4.30%Pt/FeO x -R250. Scale bar, 10 nm. ( f ) Histogram of size distributions. The circles, squares and triangles in the figures represent the single atoms, 2D rafts and 3D clusters/particles, respectively. Full size image XAFS characterization The single-atom and 2D raft structures of Pt were further characterized with extended XAFS (EXAFS) spectroscopy. As shown in Table 1 and Supplementary Fig. 6 , for the 0.08%Pt/FeO x -R200 catalyst there were a Pt-O contribution at 2.01 Å with a coordination number of 3.9 and a Pt-Fe contribution at 3.05 Å with a coordination number of 3.3. The much longer distance of Pt-Fe coordination (denoted as Pt-Fe long ) than that in Pt-Fe alloy (2.54 Å) suggests that Pt does not directly coordinate with Fe; instead, according to our previous model it coordinates with Fe via bridging oxygen [22] . The relatively higher coordination number of Pt–O (about 4) also supports this conclusion. Of most importance, there was no direct Pt–Pt coordination in this catalyst, suggesting that the Pt existed exclusively as isolated single atoms, in good agreement with the HAADF-STEM result as well as our previous observations of similar catalysts [22] . On the other hand, for the 0.08%Pt/FeO x -R250 catalyst, in addition to the Pt–O and Pt–Fe long contributions, there were also Pt–Fe and Pt–Pt long contributions at 2.55 and 2.99 Å, respectively, with a coordination number of ~1. In comparison with the 0.08% Pt/FeO x -R200 catalyst, the Pt–O coordination number in the 0.08%Pt/FeO x -R250 catalyst decreased by 50% as a consequence of elevating the reduction temperature; concurrently, the Pt–Fe metallic bonding was formed, suggesting that with the assistance of Pt, a very small portion of the Fe 3+ in the FeO x nanocrystallites was reduced to Fe 0 . Consistent with this result, the X-ray diffraction pattern of the 0.08%Pt/FeO x -R250 catalyst showed only Fe 3 O 4 phase, while that of the 0.08%Pt/FeO x -R200 catalyst presented both Fe 3 O 4 and Fe 2 O 3 phases ( Supplementary Fig. 7 ), indicating that reduction at 250 °C removed more lattice oxygen from the FeO x support. The coordination number of 1.0 for the Pt–Fe bond may suggest that on the more severe reduction treatment at 250 °C, Pt atoms moved to reside at oxygen vacancies in the FeO x support. Similar to the 0.08%Pt/FeO x -R200 catalyst, there was no Pt–Pt contribution at 2.76 Å (metallic bonding in Pt foil) in the 0.08%Pt/FeO x -R250 catalyst, while the occurrence of Pt–Pt long coordination at a distance of 2.99 Å may suggest the presence of the loosely clustered Pt single atoms as observed in the HAADF-STEM images. Therefore, the structure and behaviour of the 0.08%Pt/FeO x -R250 catalyst, in essence, resembles those of the 0.08%Pt/FeO x -R200 catalyst and therefore can be considered as a pseudo-SAC. The underlying reason for the formation of pseudo-single-atom structure is not known yet. One speculation is that the residue sodium impurity in the catalyst (from the sodium carbonate used as the precipitating agent, see Supplementary Table 1 ) may have played a role and, furthermore, sodium cations have been reported to act as a key component to stabilize the single atoms of Pt [33] . Table 1 EXAFS data fitting results of Pt/FeO x samples with different Pt loadings. Full size table With further increase of Pt loading to 0.75, 2.73 and 4.30 wt% while retaining the reduction temperature of 250 °C, the Pt–O coordination decreased while the Pt–Pt metallic bonding started to occur and then steadily increased. The Pt–Pt coordination number, however, was relatively low (0.5–2.3) for the above three catalysts, indicative of the formation of very small Pt clusters or particles. This conclusion corroborates the HAADF-STEM observations that the sizes of the majority of the Pt clusters/particles were below 1 nm, even for the 4.30%Pt/FeO x -R250 catalyst. On the other hand, the distance of Pt–Pt coordination decreased from 2.73 to 2.62 Å when the Pt loading increased from 0.75–4.30 wt%. It has been reported that the metal–metal bond distance usually contracts when the metal particles are very small [34] . However, as the percentage of isolated single atoms and pseudo-single-atom ensembles decreases with increasing Pt loading and the fact that the Pt–Pt distance in the pseudo-single-atom ensembles is much longer, the observed decrease of the Pt–Pt distance with increasing Pt loading is understandable. Thus, the EXAFS data qualitatively reflect the percentage of single-atom or pseudo-single-atom structures in the supported Pt catalysts with different Pt loadings. 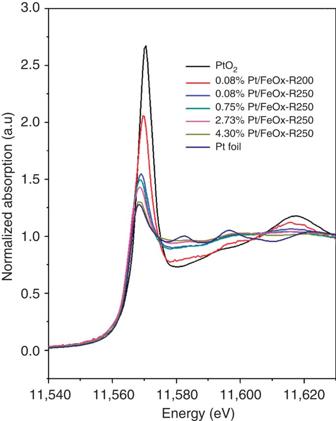Figure 2: Normalized XANES spectra at Pt LIII-edge of different Pt/FeOxsamples. The increased white-line intensity with decreasing the Pt loading indicates that single-atom and pseudo-single-atom structures of Pt are more positively charged than others. Figure 2 shows the normalized X-ray absorption near-edge structure (XANES) spectra. The white-line intensity, reflecting the oxidation state of the Pt species, increased steadily with a decrease of the Pt loading, suggesting that the Pt became more positively charged with lower Pt loading. In other words, lower Pt loading results in higher percentage of single-atom and pseudo-single-atom structures in the catalyst, and more electron transfers from Pt to the FeO x support [22] . Moreover, with the same Pt loading of 0.08 wt%, the 250 °C reduction treatment resulted in lower white-line intensity than that of the catalyst with a 200 °C reduction treatment. The changing pattern for the white-line intensity is consistent with that of the Pt–O coordination number, providing further evidence that the electronic property of Pt can be effectively tuned by forming unique nanoscale or atomic scale Pt structures. Figure 2: Normalized XANES spectra at Pt L III -edge of different Pt/FeO x samples. The increased white-line intensity with decreasing the Pt loading indicates that single-atom and pseudo-single-atom structures of Pt are more positively charged than others. Full size image By combining HAADF-STEM and XAFS techniques, the single-atom, pseudo-single-atom, as well as subnanometre and nanometre structures of Pt have been identified unequivocally. Subsequently, these catalysts with different Pt structures were tested for chemoselective hydrogenation of nitroarenes. Activity test The catalytic activity test began with the chemoselective hydrogenation of 3-nitrostyrene, the most demanding reaction among a variety of substituted nitroarenes, because the C=C group in this molecule is highly reactive towards reduction over typical Pt catalysts [6] . Before the activity tests, all the catalysts were in situ pretreated in toluene at 40 °C, 1 MPa H 2 for 1 h to remove the surface contamination by oxygen during sample handling. The reaction was conducted under a mild condition ( T =40 °C, P =3 bar) and the results are summarized in Table 2 . Over the SAC 0.08%Pt/FeO x -R200, the conversion of 3-nitrostyrene attained 95.6% within 49 min (entry 1), which was only 1/17 of the time required to achieve similar conversion level over the Pt/TiO 2 catalyst under identical conditions (entry 8). More importantly, the selectivity to 3-aminostyrene was as high as 98.4% at 95.6% conversion. The only byproduct was 3-ethylaniline and no phenylhydroxylamine was detected. Table 2 Chemoselective hydrogenation of 3-nitrostyrene on different Pt/FeO x catalysts*. Full size table As expected, the pseudo-SAC, 0.08%Pt/FeO x -R250, yielded almost the same activity and selectivity as the 0.08%Pt/FeO x -R200 SAC did, implying that both catalysts possessed the same or similar active Pt centres. By assuming that all the single/pseudo-single Pt atoms were accessible to the reactants, we estimated the TOF of both catalysts (at <20% conversion). The results showed that both catalysts gave a TOF of ~1,500 h −1 , 20-fold higher than that of the best reported catalyst Pt/TiO 2 (ref. 15 ). Moreover, when the reaction was carried out at 80 °C the TOF was as high as 11,064 h −1 , while the selectivity to 3-aminostyrene remained above 91% (entry 3, Table 2 ). In contrast, the Pt/TiO 2 was reported to give a dramatically decreased selectivity (69.7%) at 85 °C [15] . For the chemoselective hydrogenation of nitroarene, to the best of our knowledge, our SACs and pseudo-SACs are the most active and selective catalysts ever reported in literature, far outperforming all the reported catalysts, including the IB-group metals [5] , [6] , [7] , [8] , [9] , [10] , [11] , [12] , [13] , [14] , [15] and the modified Pt-group metals [20] . The kinetic studies demonstrated that no harmful intermediates such as hydroxylamine and azoxy were produced during the reaction; the only byproduct was 3-ethylaniline ( Supplementary Fig. 8 ). Control test with the bare FeO x support (either Fe 2 O 3 or Fe 3 O 4 ) under identical conditions did not show any activity at all, highlighting the critical role of the isolated Pt single atoms and pseudo-single atoms for the hydrogenation of nitroarenes. In contrast to the 0.08%Pt/FeO x SACs and pseudo-SACs, when the Pt loading was between 0.31 and 4.30 wt%, and the reduction treatment was performed at 250 °C, the resultant catalysts exhibited declined activity and selectivity with the increase of the Pt loading (entries 4–7). For example, the 4.30%Pt/FeO x -R250 catalyst gave a TOF of 762 h −1 based on the total amount of Pt and a selectivity of 92.7%. The decreased activity and selectivity should be associated with the presence of 3D particles bigger than 1 nm in diameter where Pt–Pt metallic bonding formed, which reduced the accessibility of Pt atoms on one hand and accelerated the rate of the side reaction C=C hydrogenation on the other hand. It can be found that the change in the activity and selectivity with Pt loading is consistent with that in the white-line intensity of the XANES spectra ( Fig. 2 ), suggesting that the positively charged Pt single and pseudo-single atoms should be the most active sites for the chemoselective reduction. Interestingly, the selectivity exceeding 90% achieved over the high-loading Pt catalysts (entries 6, 7) was unexpected and in remarkable contrast to the case of Pt/TiO 2 or Pt/C where a high selectivity (>90%) was only achieved with a low loading of Pt (0.2 wt%) [20] . Although the underlying reason is yet to be investigated, the FeO x support may play an important role. As shown in Table 2 , even if at a low loading of Pt (0.08 wt%), neither the Pt/SiO 2 nor the Pt/Al 2 O 3 could give rise to an acceptable chemo-selectivity (entries 9–10) in spite of the very small Pt particle sizes in those catalysts ( Supplementary Fig. 9 ). According to previous studies [11] , the nitro group in the substrate could be preferentially adsorbed on the support surface when a basic or reducible support was used. The strong interaction between the Pt single and pseudo-single atoms with the surfaces of the FeO x nanocrystallites plays an important role in determining the selectivity. To further understand the degree of the metal–support interaction, we conducted temperature-programmed reduction with H 2 (H 2 -TPR). With a decrease of Pt loading, the first peak of H 2 -TPR shifted to higher temperatures ( Supplementary Fig. 10 ), which is consistent with the XANES result that the Pt species became more positively charged with the reduction of Pt loading. Calculation of the H 2 consumption ( Supplementary Table 2 ) revealed that the first peak was not only due to the reduction of Pt(IV) but also of Fe(III) via the spillover of H 2 . The difference between the total H 2 consumption at the first peak and the H 2 consumed for Pt(IV) can be considered as an indicator of the extent of H 2 spillover; the more extensive H 2 spillover, the stronger the metal–support interaction. To provide a quantitative evaluation of the metal–support interaction, herein we define a parameter, the ratio of the moles of Fe 3+ reduced to Fe 2+ , to the moles of Pt 4+ to Pt 0 . As shown in Supplementary Table 2 , the ratio increases with a decrease of Pt loading or reduction of Pt cluster size and maximizes at 0.08 wt% Pt loading, indicating that the interaction between single or pseudo-single atoms of Pt with the FeO x support is the strongest among various Pt structures. Such strong interaction favours the chemoselective reduction of nitroarenes. In addition to the support effect, the nature of the catalytically active metal significantly affects the selectivity of the reaction. As shown in Supplementary Table 3 , the Ir 1 /FeO x SAC with an iridium loading of 0.2 wt% (see also STEM images in Supplementary Fig. 11 ) gave a conversion of 98.4% with a selectivity to 3-aminostyrene of 98.7% within 240 min, demonstrating the power of single atoms in directing the chemoselective hydrogenation. On the other hand, 0.17 wt% Pd/FeO x catalysed the complete hydrogenation of both –NO 2 and –C=C groups, resulting in a poor selectivity to 3-aminostyrene (16.0%) in spite of its high activity. The 0.17 wt% Rh/FeO x catalyst yielded only a moderate selectivity (66.1%), whereas the 0.17 wt% Au/FeO x was totally inactive under such a mild reaction condition. These extensive experimental data clearly demonstrate that with the same type of FeO x nanocrystallites as support material, different metals, even if highly dispersed, behave differently. The appropriate tuning of the metal–support interaction is essential to developing high-performance SACs. For the specific chemoselective hydrogenation of nitroarenes, Pt SACs and pseudo-SACs, among various FeO x -supported noble metals, gave the best activity and selectivity. To unveil the underlying factors that provide the superior selectivity in the chemoselective hydrogenation of nitroarenes, we performed control experiments on both the SAC 0.08%Pt/FeO x -R200 and the pseudo-SAC 0.08%Pt/FeO x -R250, with styrene and nitrobenzene as the substrates, respectively. As shown in Supplementary Table 4 , the TOFs for the hydrogenation of styrene and nitrobenzene over the 0.08%Pt/FeO x -R200 catalyst were 1,453 and 2,414 h −1 , respectively, demonstrating that the SAC was intrinsically more active for the nitrobenzene hydrogenation. In contrast, for the pseudo-SAC, the TOFs for the two reactions were comparable (2,377 h −1 versus 2,175 h −1 ). Clearly, in spite of the absence of strong Pt–Pt metallic bond in the pseudo-SAC, it was still significantly active for C=C hydrogenation due to the clustering of single atoms of Pt (formation of Pt–Pt long ) or the formation of Pt–Fe metallic bond. However, with the presence of both functional groups, that is, when a mixture (1:1) of styrene and nitrobenzene was introduced, the TOF of the pseudo-SAC for styrene hydrogenation dramatically dropped from 2,377 to 139 h −1 , while the TOF for the hydrogenation of nitrobenzene was slightly enhanced from 2,175 to 2,538 h −1 . A very similar case also occurred for the SAC. If the nitro group preferentially adsorbed on the catalyst surface, resulting significantly suppressed adsorption and the subsequent hydrogenation of the C=C bond, then the above experimental observation can be explained. Similar result was also reported on the Pt/TiO 2 catalyst [35] . In comparison with homogeneous catalysts, the most outstanding advantage of the heterogeneous catalyst is its capability for easy separation and recycling. The employment of the magnetic FeO x support allows for easy separation of the catalyst from the reaction medium, as shown in Supplementary Fig. 12 . The recovered Pt pseudo-SAC, 0.08%Pt/FeO x -R250, can be reused for at least five times without any loss of the selectivity, although the activity has a slight decay. The HAADF-STEM and XANES characterizations of the recycled catalyst ( Supplementary Figs 13–14 ) revealed that both the pseudo-single-atom structure and the oxidation state of Pt remained unchanged, demonstrating the excellent stability of the catalyst. Substrate tolerance is another important criterion to evaluate the application potential of such catalysts. Our pseudo-SAC showed good tolerance to a broad spectrum of substituted nitroarenes containing –C=C, -C=O, –C≡N and –X functional groups. In most cases, the selectivity to functionalized anilines was >97% at the nitroarene conversion level of >90% ( Table 3 ). Table 3 Chemoselective hydrogenation of different substituted nitroarenes over the 0.08%Pt/FeO x -R250 catalyst. Full size table In conclusion, we have developed highly active and chemoselective catalysts for hydrogenation of substituted nitroarenes by tuning the interactions of noble metal, especially Pt, single atoms and pseudo-single atoms with the metal oxide supports, especially FeO x nanocrystallites. The pseudo-single-atom ensembles consisting of several to tens of single atoms that are loosely associated with each other possess unique geometric and electronic properties resembling those of the SAC and provide excellent performance for the chemoselective hydrogenation reactions. Under mild reaction conditions (40 °C, 3 bar H 2 ), both the SACs and pseudo-SACs gave rise to a TOF as high as ~1,500 h −1 and a selectivity to functionalized anilines >98%, with good tolerance to substrates and excellent reusability. The superior performance of these catalysts can be attributed to strong metal–support interaction, resulting in significant electron transfer from the Pt atoms or ensembles to the FeO x support. The presence of positively charged Pt centres, the absence of Pt–Pt metallic bonding and the appropriately reduced metal oxide surfaces favour the preferential adsorption of nitro groups, leading to significantly enhanced performance. The strategy and approach discussed in this paper are general and can be extended to guide the design and development of novel catalysts for a broad spectrum of green synthesis of fine chemicals. This work also demonstrates the potential of single-atom structures in bridging homogeneous and heterogeneous catalysis. Preparation of Pt/FeO x catalysts The Pt/FeO x catalysts were prepared by co-precipitation of an aqueous solution of chloroplatinic acid (H 2 PtCl 6 ·6H 2 O, 7.59 × 10 −2 mol l −1 ) and ferric nitrate (Fe(NO 3 ) 3 ·9H 2 O, 1 mol l −1 ), with sodium carbonate at 50 °C, with the pH value of the resulting solution controlled at about 8. The recovered solid was dried at 60 °C overnight and calcined at 400 °C for 5 h. The preparation of Pd/FeO x , Rh/FeO x and Au/FeO x catalysts was similar to that of Pt/FeO x . Ir 1 /FeO x catalyst was synthesized by co-precipitation of an aqueous solution of H 2 IrCl 6 and Fe(NO 3 ) 3 with sodium hydroxide at 80 °C, with the pH value of the resulting solution controlled at about 8. The recovered solid was dried at 80 °C overnight without any further heat treatment. Pt/SiO 2 and Pt/Al 2 O 3 catalysts were prepared by incipient wetness impregnation. Pt/TiO 2 was prepared according to the literature. [20] Before characterization and reactivity test, the samples were reduced in 10% H 2 /He at 200 or 250 °C for 0.5 h. Measurements of catalytic activities The hydrogenation of nitroarenes was conducted in an autoclave equipped with pressure control system. Before the activity test, the catalyst was first put into the autoclave, to which 5 ml toluene was added, and then the autoclave was charged with 1 MPa hydrogen and heated at 40 °C for 1 h to allow for the reduction treatment of the catalyst ( Supplementary Table 5 ). After that, toluene was removed and a mixture of nitroarene substrate, toluene and internal standard O-xylene, in a total volume of 5 ml, was put into the autoclave. Next, the autoclave was flushed with 10 bar hydrogen for five times. After being sealed, the autoclave was charged with H 2 until 3 bar, then it was heated to 40 °C in a water bath with a magnetic stirrer to initiate the reaction. The H 2 pressure decreased gradually during the reaction as a result of hydrogenation. After reaction, the product was analysed by gas chromatography–mass sprctrometry. The TOF value was separately measured by keeping the substrate conversion below 20% and the calculation of the TOF was based on the total Pt loading in the catalyst. Characterization techniques The loadings of Pt were measured on inductively coupled plasma spectrometer on an IRIS Intrepid II XSP instrument (Thermo Electron Corp.). X-ray diffraction analysis was performed on a PANalytical X’ pert diffractometer equipped with a Cu Ka radiation source with a scanning angel (2 θ ) of 10–80°, operated at 40 kV and 40 mA. The H 2 -TPR was performed on an Auto Chem II 2,920 automatic catalyst characterization system (the detection limit was 5 p.p.m. H 2 ). For each measurement, ~50 mg of a catalyst was loaded into a U-shape quartz reactor and purged with He at 150 °C for 0.5 h, to remove adsorbed carbonates and hydrates. Next, after cooling to room temperature the flowing gas was switched to a 10 vol% H 2 /Ar and the catalyst was heated to 800 °C at a ramping rate of 10 °C min −1 . HAADF-STEM images were obtained on a JEOL JEM-ARM200F equipped with a CEOS probe corrector, with a guaranteed resolution of 0.08 nm. Before microscopy examination, the samples were suspended in ethanol with an ultrasonic dispersion for 5–10 min and then a drop of the resulting solution was dropped onto a holey carbon film supported by a TEM copper grid. The XAFS spectra at Pt L III -edge of the samples were measured at beamline 14 W of Shanghai Synchrotron Radiation Facility in China and beamline 17C1 of National Synchrotron Radiation Research Center in Taiwan. The output beam was selected by Si(111) monochromator. The energy was calibrated by the Pt foil. Before measurement, the samples were reduced under 10%H 2 /He at 200 or 250 °C for 0.5 h, followed by purging with pure He until cooled to room temperature. Next, the samples were evacuated and transferred to glove box without exposure to air. The sample was sealed in Kapton films in the glove box before XAFS measurement. The data were collected at room temperature under fluorescence mode by using solid state detector. Pt foil as standard compound was measured simultaneously by using the third ionization chamber so that energy calibration could be performed scan by scan. Athena software package was employed to process the EXAFS data. How to cite this article : Wei, H. et al. FeO x -supported platinum single-atom and pseudo-single-atom catalysts for chemoselective hydrogenation of functionalized nitroarenes. Nat. Commun. 5:5634 doi: 10.1038/ncomms6634 (2014).